High-resolution structure and mechanism of an F/V-hybrid rotor ring in a Na+-coupled ATP synthase All rotary ATPases catalyse the interconversion of ATP and ADP-P i through a mechanism that is coupled to the transmembrane flow of H + or Na + . Physiologically, however, F/A-type enzymes specialize in ATP synthesis driven by downhill ion diffusion, while eukaryotic V-type ATPases function as ion pumps. To begin to rationalize the molecular basis for this functional differentiation, we solved the crystal structure of the Na + -driven membrane rotor of the Acetobacterium woodii ATP synthase, at 2.1 Å resolution. Unlike known structures, this rotor ring is a 9:1 heteromer of F- and V-type c-subunits and therefore features a hybrid configuration of ion-binding sites along its circumference. Molecular and kinetic simulations are used to dissect the mechanisms of Na + recognition and rotation of this c-ring, and to explain the functional implications of the V-type c-subunit. These structural and mechanistic insights indicate an evolutionary path between synthases and pumps involving adaptations in the rotor ring. Rotary ATPases are ubiquitous membrane-bound macromolecular enzymes with similar architecture and mechanism but two distinct physiological functions. All rotary ATPases consist of a transmembrane domain, which mediates the permeation of H + or Na + , and a soluble domain, where ATP is either hydrolysed or synthesized [1] ( Supplementary Fig. 1 ). Catalysis in the soluble domain is coupled to the rotation of a sub-complex within the membrane domain, known as the c-ring, against a static, adjacent element, known as subunit-a. Viewed from the soluble domain, this rotation is clockwise when the enzyme hydrolyses ATP, leading to active ion transport. If the mechanism is instead driven by ion flow down the gradient, the c-ring rotates counter-clockwise and ATP is synthesized. Although the directionality of this rotary mechanism can be typically reversed in vitro [2] , [3] , [4] , [5] , individual enzymes are functionally specialized in vivo . F-type enzymes, in the membranes of bacteria, mitochondria and chloroplasts, function as ATP synthases [6] . A-type enzymes are also synthases, but are specific to archaea [7] . V-type enzymes, however, function as ATP-driven ion pumps in eukaryotic vacuolar membranes [8] . This physiological specialization suggests that structural adaptations might have evolved to optimize a given functionality. A long-standing hypothesis is that the c-subunits that constitute the rotor ring might contribute to this differentiation [9] . Prototypical c-rings of bacterial and eukaryotic ATP synthases are homomers of c-subunits with a simple topology, namely a hairpin of two transmembrane helices [10] , [11] , [12] , [13] , [14] ( Supplementary Fig. 2 ). The number of c-subunits assembled varies across species (from 8 to 15 to date [15] , [16] ), but canonical F-type c-rings consistently feature an uninterrupted series of ion-binding sites along their outer circumference, each located at the interface between two adjacent hairpins, approximately halfway across the membrane. The prototypical c-rings of ATP-driven pumps, however, typically consist of c-subunits with double hairpins [17] , presumably resulting from gene duplications [18] . Intriguingly, these rings usually feature fewer ion-binding sites due to mutation of key amino acids required for ion coordination ( Supplementary Fig. 2 ). Moreover, some eukaryotic V-type c-rings seem to consist of c-subunits with different amino acid sequence. For example, the c-ring of the vacuolar ATPase of Saccharomyces cerevisiae appears to be a heteromer of three different double-hairpin c-subunits (c, c’, c’’), although its stoichiometry remains unclear [19] , [20] , [21] . To begin to rationalize how the evolution of the c-ring may have contributed to the functional specialization of different rotary ATPase subfamilies, we isolated the c-ring from the F-type ATP synthase of A. woodii and solved its structure by X-ray crystallography. Consistent with previous biochemical studies [22] , we find that this c-ring consists of a combination of prototypical F- and V-type c-subunits, thus resembling an evolutionary intermediate. The structure provides the basis for molecular and kinetic simulations, through which we examine the mechanistic and thermodynamic implications of this unprecedented hybrid stoichiometry. Structure of the A. woodii c-ring The crystal structure of the c-ring from the A. woodii ATP synthase was resolved at 2.1 Å resolution ( Supplementary Fig. 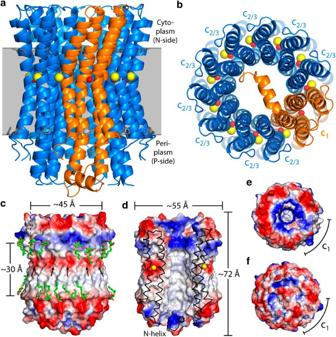Figure 1: Structure of the heteromeric c-ring from theAcetobacterium woodiiATP synthase. The ring is viewed (a) along the membrane plane and (b) from the periplasm, highlighting the two c-subunit topologies (blue and orange cartoons), as well as the bound Na+ions (yellow spheres) and the co-coordinating water molecules (red spheres). Note the site within subunit c1does not bind Na+. Residues L55/F77 in c2/3and L72/L155/F94/Y177 in c1indicate the probable position of the ring within the membrane (grey). (c) Electrostatic potential at the outer surface of the c-ring and (d) at the surface of the central hydrophobic pore. Detergent molecules (green) resolved in the electron density map are highlighted. Arrows indicate the position of the ion-binding sites. (e) Asymmetry of the electrostatic potential on the cytoplasmic face of the c-ring, where the central stalk binds. (f) The N-terminal extension of subunit c1occludes the central pore almost completely. 3 and Supplementary Table 1 ). Consistent with our previous biochemical analysis [22] , the ring is an assembly of nine copies of single-hairpin c-subunits, referred to as c 2/3 , and one copy of a double-hairpin c-subunit, or c 1 ( Fig. 1a,b ). Thus, the structure consists of 22 transmembrane α-helices, arranged in two concentric, staggered rings of 11 helices each. The c-ring is ~72 Å in height and is shaped similar to an hourglass with a central pore perpendicular to the membrane plane ( Fig. 1 ). The outermost diameter is widest (~55 Å) on the cytoplasmic and periplasmic sides, and is narrowest approximately halfway across the membrane (~45 Å). In the c 2/3 subunits, the amino-terminal (or inner) helix and the carboxy-terminal (or outer) helix are connected on the cytoplasmic side by a short, rigid loop, which mediates crystal contacts ( Supplementary Fig. 4 ). The c 2/3 subunits are structurally very similar (root mean square deviation (r.m.s.d. )<1 Å) to other F-type single-hairpin c-subunits ( Supplementary Fig. 5 ), particularly those in the Ilyobacter tartaricus c 11 ring [12] (r.m.s.d.~0.4 Å). Figure 1: Structure of the heteromeric c-ring from the Acetobacterium woodii ATP synthase. The ring is viewed ( a ) along the membrane plane and ( b ) from the periplasm, highlighting the two c-subunit topologies (blue and orange cartoons), as well as the bound Na + ions (yellow spheres) and the co-coordinating water molecules (red spheres). Note the site within subunit c 1 does not bind Na + . Residues L55/F77 in c 2/3 and L72/L155/F94/Y177 in c 1 indicate the probable position of the ring within the membrane (grey). ( c ) Electrostatic potential at the outer surface of the c-ring and ( d ) at the surface of the central hydrophobic pore. Detergent molecules (green) resolved in the electron density map are highlighted. Arrows indicate the position of the ion-binding sites. ( e ) Asymmetry of the electrostatic potential on the cytoplasmic face of the c-ring, where the central stalk binds. ( f ) The N-terminal extension of subunit c 1 occludes the central pore almost completely. Full size image The c 1 subunit consists of four transmembrane helices and thus resembles a prototypical V-type c-subunit. The first and third helices are part of the inner ring, while the second and fourth face the lipid bilayer ( Fig. 1a,b ). An unusual α-helical extension at the N-terminus of the c 1 subunit is also well resolved, projecting across the central pore towards a distal c 2/3 subunit, parallel to the membrane plane. The loop that connects the two hairpins in c 1 on the periplasmic side, which is significantly longer than the cytoplasmic loops within each of the hairpins, can be clearly discerned too. Aside from these two features, the structure of c 1 is nearly identical to that of two adjacent c 2/3 subunits (r.m.s.d.~0.3 Å) ( Supplementary Fig. 5 ), and is also similar to the double-hairpin c-subunit of the V-type ATPase from Enterococcus hirae [17] (r.m.s.d.<2 Å). The membrane-exposed face of the c-ring is primarily hydrophobic ( Fig. 1c ); neighbouring electron densities probably correspond to bound detergent molecules, marking the boundaries of the lipid bilayer (~30 Å) ( Fig. 1c ). The surface of the central pore is also highly hydrophobic ( Fig. 1d ) and residual electron densities visible therein seem to also originate from disordered detergent molecules. The pore diameter is ~17 Å at its narrowest and the length of the hydrophobic region is ~30 Å. Thus, in native membranes this pore is probably occluded by a lipid bilayer formed by a handful of molecules, slightly shifted towards the periplasm. The periplasmic and cytoplasmic sides of the c-ring are rich in charged and polar amino acids ( Fig. 1e,f ). The cytoplasmic surface is largely electronegative, due to a glutamate residue in the cytoplasmic loop of the c 2/3 subunits (sequence RQPE) ( Fig. 1e,f and Supplementary Fig. 2 ). Interestingly, the two hairpin loops in the c 1 subunit (of sequence KNPT and IRPE, respectively) alter this pattern, and the surface here is electropositive, which may enhance the interaction of the c-ring with subunits γ and ε. In F-type ATP synthases, these subunits form a sub-complex referred to as the central stalk, which is essential to mechanically couple the ion-conducting and catalytic domains. On the periplasmic side, the N-terminal helix in the c 1 subunit occludes the central pore almost completely ( Fig. 1f ). Nevertheless, small openings between this helix and the inner pore wall remain, which could conceivably allow passage of protons, ions or water. It is thus likely to be that the pore is actually sealed by lipid molecules, as observed in other rings [23] , [24] , [25] , so as to prevent the dissipation of the electrochemical gradient across the membrane. The Na + -binding sites in the A. woodii c-ring The A. woodii c-ring features a series of Na + -binding sites on its lipid-exposed outer surface, close to the membrane centre ( Fig. 1a,b ). Specifically, binding sites occupied by Na + can be clearly discerned at each of the eight interfaces between single-hairpin c 2/3 subunits, sandwiched between the two outer helices, as well as at the two interfaces between c 2/3 and c 1 subunits ( Fig. 2a,b,d ). Na + is electrostatically stabilized by a glutamate side chain, located in the outer helix of one of the flanking c-subunits. A carboxylate group at this position is conserved in all known c-ring binding sites, both in enzymes coupled to Na + (refs 12 , 17 , 26 ) as well as those coupled to H + , which bind to the c-ring by protonation [13] , [14] , [27] , [28] . Three other protein groups coordinate the ion: a glutamine carbonyl, from the inner helix of the same subunit as the key glutamate, and a threonine hydroxyl and a backbone carbonyl, from the outer helix of the adjacent subunit ( Fig. 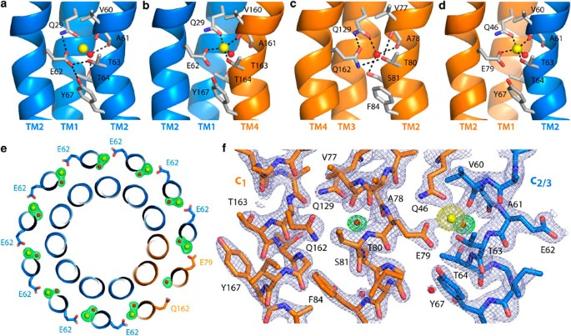Figure 2: Configuration of ion-binding sites in theA. woodiic-ring. (a) One of the eight Na+-binding sites at the interfaces between c2/3subunits, viewed from the membrane. The protein residues (grey sticks) and water molecule (red sphere) coordinating the ion (yellow sphere) are highlighted. (b) The Na+-binding site at the c2/3/c1interface. (c) The water-binding site within the c1subunit. (d) The Na+-binding site at the c1/c2/3interface. Dashed lines indicate inferred hydrogen bonds inaandcand ion–protein contacts inbandd. (e)Fo−Fcdifference map (green mesh) for all bound Na+and water molecules, contoured at +5.0σ. The ring is viewed from the cytoplasmic side. (f)Fo−Fcmaps for either Na+or water molecules (yellow and green mesh, respectively) bound within c1and the c1/c2/3interface, contoured at +4.0σ. The 2Fo−Fcmap for the protein is also shown, contoured at 2.4σ(light blue mesh).Supplementary Fig. 6shows a stereo view of this figure. 2 and Supplementary Table 2 ). Consistent with other structures of Na + -coupled c-rings [26] , [29] , a bound water molecule co-coordinates Na + in all sites ( Fig. 2 and Supplementary Table 2 ). This ion-coordination network is stabilized by several peripheral side chains; for example, hydrogen bonds can be inferred between the key glutamate and a tyrosine, and between the bound water molecule and a threonine ( Fig. 2a,b,d ). Although this motif is chemically selective for protons [30] , [31] , the much larger amount of sodium ions over protons in the crystallization buffer (100 mM Na + and pH 4.5) ensures Na + binding. This concentration effect is also present physiologically, and hence this crystal structure confirms earlier functional measurements indicating that ATP synthesis in A. woodii is driven directly by a sodium-motive force [32] . Figure 2: Configuration of ion-binding sites in the A. woodii c-ring. ( a ) One of the eight Na + -binding sites at the interfaces between c 2/3 subunits, viewed from the membrane. The protein residues (grey sticks) and water molecule (red sphere) coordinating the ion (yellow sphere) are highlighted. ( b ) The Na + -binding site at the c 2/3 /c 1 interface. ( c ) The water-binding site within the c 1 subunit. ( d ) The Na + -binding site at the c 1 /c 2/3 interface. Dashed lines indicate inferred hydrogen bonds in a and c and ion–protein contacts in b and d . ( e ) F o − F c difference map (green mesh) for all bound Na + and water molecules, contoured at +5.0 σ . The ring is viewed from the cytoplasmic side. ( f ) F o − F c maps for either Na + or water molecules (yellow and green mesh, respectively) bound within c 1 and the c 1 /c 2/3 interface, contoured at +4.0 σ . The 2 F o − F c map for the protein is also shown, contoured at 2.4 σ (light blue mesh). Supplementary Fig. 6 shows a stereo view of this figure. Full size image Interestingly, the potential binding site at the interface between the two hairpins within the c 1 subunit lacks a Na + ion ( Fig. 2c,e,f and Supplementary Fig. 6 ). This site is rich in polar groups and a water molecule can be clearly discerned in the electron density map, forming hydrogen bonds with the protein ( Fig. 2c,f ). However, no density for Na + was detected, despite the high Na + concentration in the crystallization buffer. This is due to the substitution of the prototypical carboxyl side chain by glutamine (Gln162); because of its neutral charge, the carboxamide group cannot offset the cost of Na + dehydration upon binding to a site immersed in a mostly hydrophobic environment (that is, detergent in the crystal). We conclude, therefore, that in a complete revolution the A. woodii c-ring transports ten ions across the membrane. Direct visualization of the c-ring by AFM The N-terminal α-helical extension of the c 1 subunit is ~20 amino acids in length and partially hydrophobic. In the crystal structure, this helix lies across the central pore rather than being inserted in the membrane ( Fig. 1b ). To assess whether this is the native conformation, we studied a series of two-dimensional arrays of A. woodii c-rings via atomic force microscopy (AFM), in a physiological buffer and at room temperature (RT) ( Fig. 3a ). We specifically analysed the periplasmic face of the c-ring via single-particle classification and averaging (Methods). The resulting five class-averages consistently show ten identical density peaks along the c-ring circumference, followed by a depression ( Fig. 3b,c and Supplementary Fig. 7 ). Adjacent to it, in the clock-wise direction, a rod-like density projects across the central pore of the ring, in an orientation that is similar in all class averages. This rod is the highest object in the density, particularly in close proximity to its distal end ( Fig. 3d,e ). All these features are consistent with the crystal structure: the regular pattern of densities along the ring circumference corresponds to the elongated N-termini of the c 2/3 subunits, which protrude from the membrane; the depression in this pattern is the loop connecting the two c 1 subunit hairpins, which protrudes less than the c 2/3 N-termini; and lastly, the rod projecting across the pore is the N-terminal extension of the c 1 subunit. Thus, the AFM data confirms both the 9c 2/3 :1c 1 stoichiometry of the A. woodii c-ring and the conformation of the c 1 N-terminal α-helix observed in the crystal structure. 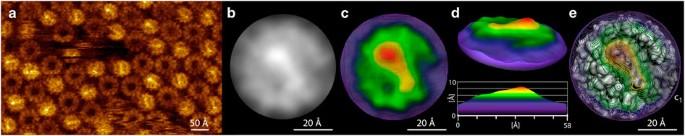Figure 3: High-resolution AFM of theA. woodiic-ring. (a) Topograph ofA. woodiic-rings densely reconstituted in a lipid membrane22(reproduced with kind permission from the publisher). (b) Representative class-average of the periplasmic face of the c-ring from single-particle analysis (see alsoSupplementary Fig. 7). (c) Density data calculated fromb, coloured according to height. (d) Same data as inc, viewed diagonally and in cross-section. (e) Same data as inc, contoured and overlaid on the molecular surface of the c-ring. The position of subunit c1is indicated. Figure 3: High-resolution AFM of the A. woodii c-ring. ( a ) Topograph of A. woodii c-rings densely reconstituted in a lipid membrane [22] (reproduced with kind permission from the publisher). ( b ) Representative class-average of the periplasmic face of the c-ring from single-particle analysis (see also Supplementary Fig. 7 ). ( c ) Density data calculated from b , coloured according to height. ( d ) Same data as in c , viewed diagonally and in cross-section. ( e ) Same data as in c , contoured and overlaid on the molecular surface of the c-ring. The position of subunit c 1 is indicated. Full size image The role of this α-helical extension is, however, not apparent. Given its conformation, it is unlikely to be directly involved in the mechanism of the enzyme. A reasonable speculation is that it contributes to make c-rings with a 9c 2/3 :1c 1 stoichiometry more statistically abundant than those with a greater number of c 1 subunits. In previous studies of the factors controlling c-ring assembly, we have shown that several stoichiometries co-exist in equilibrium, albeit one form is thermodynamically dominant, particularly for native amino acid sequences [5] , [33] . As the observed conformation of this amphipathic helix is sterically possible only if the ring contains one c 1 subunit, other oligomeric states (for example, 7c 2/3 :2c 1 ) would necessarily expose a large hydrophobic surface to water, and hence be energetically disfavoured. Mechanism of Na + loading and release The ion-locked conformation of the Na + -binding sites in the structure of the A. woodii c-ring ( Fig. 2 ) is very similar to that observed in other high-resolution c-ring structures resolved using detergent-based crystallization buffers [12] , [13] , [17] , [26] , [28] . We have previously shown, for a H + -coupled c-ring, that this is the configuration of the sites that face the membrane during the enzyme’s rotary cycle [34] . The p K a of these sites is highly elevated, and thus they do not exchange protons with the bulk solution. Proton loading and release, either downhill or uphill, takes place instead when the sites become sequentially exposed to the adjacent subunit-a as the c-ring rotates around its axis [35] , [36] . The atomic structure of subunit-a is to date unknown, but cysteine-accessibility measurements have indicated that this subunit and/or its interface with the c-ring feature two aqueous channels that reach the c-ring ion-binding sites from either side of the membrane [37] . Our previous analysis showed that this hydrated micro-environment facilitates proton exchange by triggering a local conformational change in the binding sites, and by shifting down their p K a [34] . Specifically, hydration causes the key glutamate side chain to adopt an exposed outward orientation that facilitates reversible deprotonation, without the need of a competing electrostatic interaction. This proposal was recently validated by high-resolution structures of a mitochondrial H + -coupled c-ring, solved using a detergent-free crystallization buffer primarily consisting of 2-methyl-2,4-pentanediol (MPD) in water [14] . This amphiphilic compound coats the hydrophobic surface of the c-ring, but unlike detergent it permits the H + -binding sites to be hydrated [14] . Accordingly, the binding sites in the mitochondrial c-ring structure adopt the predicted unlocked conformation [34] and can become deprotonated [14] . To assess whether this mechanism applies to the A. woodii ATP synthase and other Na + -coupled ATPases, we carried out a series of molecular dynamics (MD) simulations of the A. woodii c-ring solubilized in an MPD/water buffer ( Supplementary Figs 8 and 9 ). Spontaneous Na + dissociation events were indeed observed in independent simulations, after 100–200 ns ( Fig. 4a ). The mechanism of Na + unloading is very similar to that proposed previously for H + ( Fig. 4b and Supplementary Movie 1 ). The Na + ion exits the binding site along with the key glutamate, as this side chain rotates outwards in what appears to be a thermal fluctuation. As water molecules gradually penetrate the binding site, disrupting the network of hydrogen-bonding interactions therein, Na + remains transiently bound to the carboxyl group, but on formation of a complete water-coordination shell the ion diffuses away, while the glutamate side chain continues to project towards the solvent. 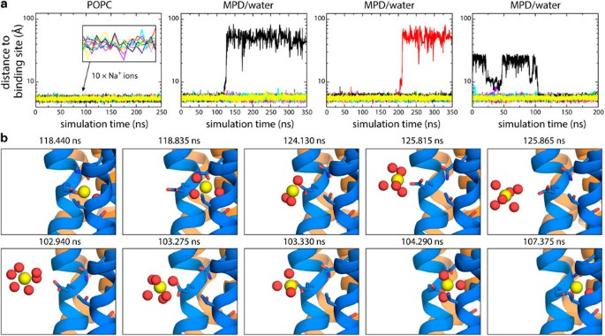Figure 4: Spontaneous unbinding and rebinding of Na+from/to theA. woodiic-ring in molecular dynamics simulations. (a) Time series of the distance between each of the ten Na+ions bound to theA. woodiic-ring and the neighbouring inner helix (residue Pro25 in c2/3subunits, or Pro42 in c1), in three independent simulations in which the ring is either embedded in a phospholipid membrane (Supplementary Fig. 8), or solubilized in 30% MPD/water (Supplementary Figs 8 and 9) (two simulations), representing the two different micro-environments of the ion-binding sites as the c-ring rotates against subunit-a. The time trace for each ion is coloured differently. (b) Representative simulation snapshots during the unbinding (upper panels) and rebinding reactions (lower panels) reveal the atomic mechanism of Na+recognition and release. The time stamp for each snapshot is indicated. Note that the configuration of the unbound site before Na+rebinding is uncorrelated from that immediately after Na+release (Supplementary Fig. 9). The c-ring is coloured as inFig. 1. Side chains and water molecules (sticks and red spheres, respectively) coordinating Na+(yellow spheres) are highlighted. Hydrogen atoms, other protein side chains and buffer molecules are omitted for clarity. Figure 4: Spontaneous unbinding and rebinding of Na + from/to the A. woodii c-ring in molecular dynamics simulations. ( a ) Time series of the distance between each of the ten Na + ions bound to the A. woodii c-ring and the neighbouring inner helix (residue Pro25 in c 2/3 subunits, or Pro42 in c 1 ), in three independent simulations in which the ring is either embedded in a phospholipid membrane ( Supplementary Fig. 8 ), or solubilized in 30% MPD/water ( Supplementary Figs 8 and 9 ) (two simulations), representing the two different micro-environments of the ion-binding sites as the c-ring rotates against subunit-a. The time trace for each ion is coloured differently. ( b ) Representative simulation snapshots during the unbinding (upper panels) and rebinding reactions (lower panels) reveal the atomic mechanism of Na + recognition and release. The time stamp for each snapshot is indicated. Note that the configuration of the unbound site before Na + rebinding is uncorrelated from that immediately after Na + release ( Supplementary Fig. 9 ). The c-ring is coloured as in Fig. 1 . Side chains and water molecules (sticks and red spheres, respectively) coordinating Na + (yellow spheres) are highlighted. Hydrogen atoms, other protein side chains and buffer molecules are omitted for clarity. Full size image To investigate the process of ion loading, a third simulation was initiated about 50 ns after a Na + unbinding event. After another ~100 ns, we observed spontaneous, uncorrelated rebinding of the ion, via a mechanism that is analogous to that of the unbinding events, but in reverse ( Fig. 4 , Supplementary Movie 2 and Supplementary Fig. 10 ). That is, the key glutamate recognizes the ion as its water-coordination sphere becomes depleted. Next the carboxyl–ion pair enters the binding site expelling most of the water therein. In the final bound state, only the water molecule that co-coordinates the ion in the experimental crystal structure remains in the site, exactly in the same location. In summary, these simulations show that Na + loading and release from the c-ring entails localized conformational changes in the binding sites. As we showed previously for protons [34] , Na + release is facilitated by hydration and does not require a competing ionic interaction, for example, between the key glutamate and subunit-a. Likewise, empty binding sites do not require a stabilizing ionic interaction to remain in a configuration suitable for Na + recognition; local hydration is sufficient. It should be noted that comparable simulations of the A. woodii c-ring in a phospholipid membrane revealed no dissociation events ( Fig. 4a and Supplementary Fig. 8 ). Dynamics of the c 1 site in response to hydration The simulations just described also provide insights into the dynamics of the site within the c 1 subunit that lacks a bound Na + . In the crystal structure, this site adopts a conformation akin to that observed in the proton-binding sites of several H + -dependent c-rings [13] , [28] , [38] . Specifically, the glutamine (Gln162) that replaces the prototypical glutamate is locked in position by several hydrogen bonds with neighbouring side chains (Gln129 and Thr80), as well as with a bound water molecule. In simulations of the c-ring in a phospholipid bilayer, this locked configuration was indeed the most frequently observed ( Fig. 5a,c ). In the MPD/water buffer, however, the locked conformation is in equilibrium with a range of configurations in which the H-bonding network in the site is disrupted by water molecules and Gln162 projects out into the solvent ( Fig. 5b,c ). These results indicate that on entering the subunit-a interface, the dynamic response of the c 1 site resembles that of the ion-binding sites in this and other c-rings [34] . It is worth noting that the c 1 site does not bind Na + even in this hydrated environment. Additional simulations in which a Na + ion is carefully modelled into the c 1 site (Methods and Fig. 5d ) consistently show immediate dissociation, in the ~10 ns time scale ( Fig. 5e ). This dissociation rate is much faster than what we observe for the actual Na + -binding sites, that is, microsecond time scale or longer (note Fig. 4a shows single dissociation events out of ten possible), indicating the Na + affinity of the c 1 site is several orders of magnitude weaker. 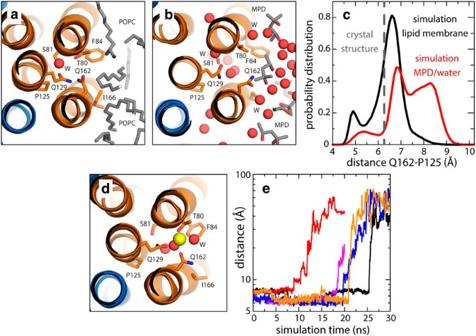Figure 5: Dynamics of the water-binding site in the V-type c1subunit. (a) Close-up of the c1site, viewed from the cytoplasm, in a representative snapshot of the simulation of the c-ring in a phospholipid membrane (Supplementary Fig. 8). The configuration closely resembles the locked conformation observed in the crystal structures of H+-dependent c-ring in detergent. (b) Close-up of the c1site in a representative snapshot of the simulation of the c-ring in the MPD/water buffer (Supplementary Figs 8 and 9). Polar interactions with the buffer unlock the H-bonding interaction network within the site, allowing Gln162 to project away into the solvent. The c-ring is represented as inFig. 1. Side chains and water molecules in the site, as well as neighbouring lipid tails or MPD molecules, are highlighted (sticks, spheres). Hydrogen atoms as well as other protein side chains and lipid head groups are omitted for clarity. (c) Probability distributions of the distance between the carboxamide group of Gln162 and Pro125, in the neighbouring inner helix, in either simulation, demonstrate the propensity of the c1site to adopt an open conformation in the hydrated environment. (d) Hypothetical configuration of the c1site with a bound Na+, equilibrated through restrained molecular dynamics simulations. Note the ion is penta-coordinated, as in the actual Na+-binding sites. (e) Rapid, spontaneous dissociation of the Na+ion modelled in the c1site in five independent simulation trajectories. Figure 5: Dynamics of the water-binding site in the V-type c 1 subunit. ( a ) Close-up of the c 1 site, viewed from the cytoplasm, in a representative snapshot of the simulation of the c-ring in a phospholipid membrane ( Supplementary Fig. 8 ). The configuration closely resembles the locked conformation observed in the crystal structures of H + -dependent c-ring in detergent. ( b ) Close-up of the c 1 site in a representative snapshot of the simulation of the c-ring in the MPD/water buffer ( Supplementary Figs 8 and 9 ). Polar interactions with the buffer unlock the H-bonding interaction network within the site, allowing Gln162 to project away into the solvent. The c-ring is represented as in Fig. 1 . Side chains and water molecules in the site, as well as neighbouring lipid tails or MPD molecules, are highlighted (sticks, spheres). Hydrogen atoms as well as other protein side chains and lipid head groups are omitted for clarity. ( c ) Probability distributions of the distance between the carboxamide group of Gln162 and Pro125, in the neighbouring inner helix, in either simulation, demonstrate the propensity of the c 1 site to adopt an open conformation in the hydrated environment. ( d ) Hypothetical configuration of the c 1 site with a bound Na + , equilibrated through restrained molecular dynamics simulations. Note the ion is penta-coordinated, as in the actual Na + -binding sites. ( e ) Rapid, spontaneous dissociation of the Na + ion modelled in the c 1 site in five independent simulation trajectories. Full size image Directionality and mechanism of c-ring rotation The directionality of the rotary mechanism of ATPases can be fully rationalized using the two-channel model mentioned earlier [35] , [36] . This model postulates (i) that the aqueous pathways across the a/c complex are two discontinuous half channels, each open to one side of the membrane and (ii) that these channels reach to two adjacent binding sites in the c-ring, such that the site exposed to the N-side of the membrane (that is, with negative electrochemical potential), which we refer to as S N , is located clockwise (as viewed from F 1 ) relative to the site exposed to the P-side (that is, with positive electrochemical potential), or S P . An additional and crucial assumption is that ions must not be able to transfer directly from S P to S N , or vice versa . Instead, an ion that binds, for example, to S P , would reach S N only when the c-ring makes a near-complete revolution, counter clockwise. A conserved arginine residue in subunit-a, proximal to the c-ring ion-binding sites [39] , is thought to interact with the conserved glutamate/aspartate in the c-subunits and to be an important element in this mechanism [40] , [41] . Although it is often imagined that this interaction is a necessary trigger for ion release from the c-ring, the calculations presented above and elsewhere [14] , [34] indicate that this is not so; a hydrated microenvironment is in fact sufficient to induce the release of ions from the c-ring. Consistent with this notion, functional assays of the Escherichia coli ATP synthase have demonstrated that neutralizing mutations of the subunit-a arginine do not preclude downhill ion diffusion across the a/c complex; the mutations, however, abolish the coupling between ion permeation and catalysis, that is, impair the rotary mechanism of the enzyme [41] , [42] . What then is the role of the conserved arginine in subunit-a? In our version of the two-channel model, depicted in Fig. 6 , the role of this side chain is to sequester one of the two binding sites at the a/c interface, already in the ion-free state, so as to preclude direct ion hopping between them. Thus, an ion that binds to S P from the P-side, while S N is engaged by the arginine, would not be able to hop directly to S N and thus leak through the N-channel; conversely, an ion that exits S N , while S P is engaged, would be necessarily released on the N-side of the membrane, and not via the P-channel. 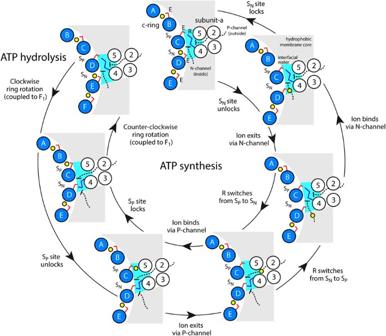Figure 6: Proposed microscopic mechanism of c-ring rotation coupled to ion transport. The diagram shows the interface between the c-ring, represented by five of the outer helices (blue circles), and subunit-a, in the topology of TM2–TM5 (white circles) predicted by cross-linking data64. Two aqueous half-channels mediate ion exchange across the a/c complex with either the P-side (outside) or the N-side (inside) of the energized membrane (black dashed lines). Hydration of the c-ring binding sites (SPand SN, respectively) facilitates loading and release of ions (yellow spheres) via isomerization of a conserved glutamate/aspartate (E, red sticks). A conserved arginine in subunit-a (R, blue sticks) forms alternating salt bridges with SPand SN, and thus prevents the ion from hopping between these sites, that is, it effectively provides an electrostatic barrier between the P and N channels. The directionality of the mechanism is thus imposed by the clockwise arrangement of SPand SNsites: downhill ion permeation (that is, from P to N) necessarily implies counter-clockwise c-ring rotations (powering ATP synthesis), while clockwise rotations (driven by ATP hydrolysis) imply uphill transport (that is, from N to P). Figure 6: Proposed microscopic mechanism of c-ring rotation coupled to ion transport. The diagram shows the interface between the c-ring, represented by five of the outer helices (blue circles), and subunit-a, in the topology of TM2–TM5 (white circles) predicted by cross-linking data [64] . Two aqueous half-channels mediate ion exchange across the a/c complex with either the P-side (outside) or the N-side (inside) of the energized membrane (black dashed lines). Hydration of the c-ring binding sites (S P and S N , respectively) facilitates loading and release of ions (yellow spheres) via isomerization of a conserved glutamate/aspartate (E, red sticks). A conserved arginine in subunit-a (R, blue sticks) forms alternating salt bridges with S P and S N , and thus prevents the ion from hopping between these sites, that is, it effectively provides an electrostatic barrier between the P and N channels. The directionality of the mechanism is thus imposed by the clockwise arrangement of S P and S N sites: downhill ion permeation (that is, from P to N) necessarily implies counter-clockwise c-ring rotations (powering ATP synthesis), while clockwise rotations (driven by ATP hydrolysis) imply uphill transport (that is, from N to P). Full size image To evaluate this key element of the mechanism, we calculated the free-energy cost associated with the transfer of a Na + ion from a loaded binding site in the A. woodii c-ring (that is, S P ) to an adjacent empty site, clockwise (that is, S N ), in which the exposed carboxyl group is paired with a guanidinium ion (GND + ), modelled in so as to mimic the interaction with the conserved arginine on subunit-a ( Fig. 7a,b ). The resulting free-energy value was ~9 kcal mol −1 ( Fig. 7c ). That is, an ion reaching S P through the P-channel would be more than a million times more likely to remain in S P than to hop to S N . Ion hopping would be also far less probable than the alternative next step in the proposed cycle, namely the rotational displacement of the c-ring ( Fig. 6 ). The energy cost of this rotational displacement is ~3 kcal mol −1 , that is, three times the free energy cost of ATP synthesis at typical ATP/ADP/P i concentrations (~11 kcal mol −1 ), distributed over 11 steps. Direct ion hopping between the two c-ring binding sites exposed at the a/c interface is therefore extremely improbable, from a purely thermodynamic standpoint (that is, even if we neglect kinetic barriers). This electrostatic separation between the P- and N-channel ensures strict coupling between ion permeation and c-ring rotation. 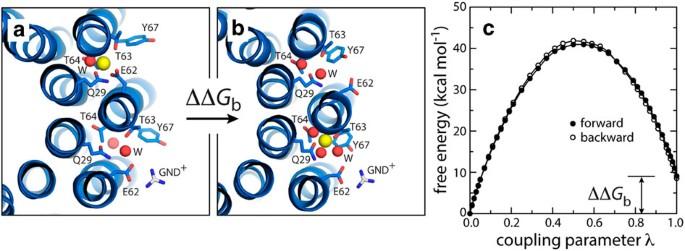Figure 7: Electrostatic barrier between the P and N channels. (a) A snapshot was extracted from one of the simulations in which Na+is spontaneously released (Fig. 5) and the exposed glutamate side chain was paired to a guanidinium ion (GND+), modelled in to represent the interaction with the key arginine side chain on TM4 of subunit-a. (b) The free-energy cost of transferring a bound Na+from the adjacent site, counter-clockwise, to the site engaged to the GND+ion was then computed by gradually decoupling the ion from its environment in configuration (a) and re-coupling it in configuration (b). (c) Free-energy change as a function of the (de)coupling parameterλ. The transfer free energy was calculated in both directions. The c-ring is represented as inFig. 1. Side chains and water molecules in the site are highlighted (sticks, spheres). Hydrogen atoms as well as other protein side chains and all MPD/water molecules are omitted for clarity. Figure 7: Electrostatic barrier between the P and N channels. ( a ) A snapshot was extracted from one of the simulations in which Na + is spontaneously released ( Fig. 5 ) and the exposed glutamate side chain was paired to a guanidinium ion (GND + ), modelled in to represent the interaction with the key arginine side chain on TM4 of subunit-a. ( b ) The free-energy cost of transferring a bound Na + from the adjacent site, counter-clockwise, to the site engaged to the GND + ion was then computed by gradually decoupling the ion from its environment in configuration ( a ) and re-coupling it in configuration ( b ). ( c ) Free-energy change as a function of the (de)coupling parameter λ . The transfer free energy was calculated in both directions. The c-ring is represented as in Fig. 1 . Side chains and water molecules in the site are highlighted (sticks, spheres). Hydrogen atoms as well as other protein side chains and all MPD/water molecules are omitted for clarity. Full size image Energetics of the arginine-switch step A necessary step in the microscopic mechanism proposed in Fig. 6 requires the key arginine side chain in subunit-a to switch between two competing interactions with the glutamate side chains in the c-ring that are exposed to the a/c interface, S P and S N . Whether or not this hypothetical step is plausible from an energetic standpoint remains to be qualified. For the A. woodii ring in particular, it is unclear whether the glutamine side chain in the V-type c 1 subunit is a viable interaction partner. To address these questions, we first designed a free-energy calculation in which a GND + ion reversibly exchanges between two adjacent Na + sites in empty c 2/3 subunits; that is, the glutamate side chains in these sites project out into the MPD/water buffer and form competing ion pairs with GND + in the course of the simulation. These two states are not structurally symmetric, but nevertheless our calculations show they are equivalent energetically ( Fig. 8a ). More surprisingly, the calculations reveal that the energy barrier between them is only ~4 kcal mol −1 (comparable to, for example, the isomerization of a single carbon–carbon bond in a linear alkane chain). Analysis of the simulated exchanges reveals this energetic penalty is small because in the transition state the GND + ion remains indirectly engaged to both carboxylate groups via ordered layers of water molecules ( Fig. 8a and Supplementary Fig. 11a ). Thus, hydration at the a/c interface not only facilitates ion release from the c-ring binding sites, but also eases the exchange between consecutive c-subunit/subunit-a interactions. 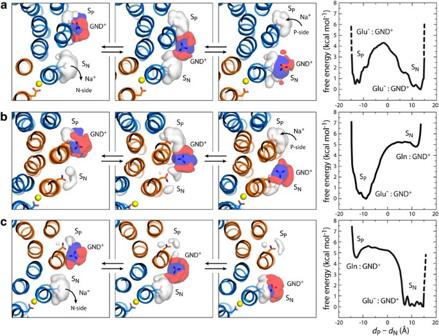Figure 8: Energetics of exchange of sequential subunit-a/subunit-c interactions in the rotary cycle. The interaction of the c-subunits with the key arginine on subunit-a was again mimicked with a GND+ion (grey/blue sticks) added to the MPD/water buffer. (a) GND+exchange between two unlocked glutamate side chains (blue sticks) in adjacent Na+-binding sites, that is, after Na+release from the SNsite and before Na+loading to the SPsite. The three panels on the left depict the end-point states in the exchange and the transition state in between. The coloured volumes are density maps extracted from the simulations, mapping the location of either GND+(blue), the first hydration shell of GND+(red), or the first hydration shell of the carboxylate groups (white). Representative snapshots are shown inSupplementary Fig. 11. The panel on the right shows the free-energy profile associated with the exchange, as a function of the distances between the GND+ion and SPand SN(dPanddN). A two-dimensional free-energy surface is shown inSupplementary Fig. 11. (b) Exchange between the unlocked glutamine side chain in the c1subunit (orange sticks) and the glutamate side chain in the adjacent Na+site, counter-clockwise. (c) Same asb, clockwise. The c-ring is represented as inFig. 2. Hydrogen atoms as well as protein side chains and MPD/water molecules are omitted for clarity. Figure 8: Energetics of exchange of sequential subunit-a/subunit-c interactions in the rotary cycle. The interaction of the c-subunits with the key arginine on subunit-a was again mimicked with a GND + ion (grey/blue sticks) added to the MPD/water buffer. ( a ) GND + exchange between two unlocked glutamate side chains (blue sticks) in adjacent Na + -binding sites, that is, after Na + release from the S N site and before Na + loading to the S P site. The three panels on the left depict the end-point states in the exchange and the transition state in between. The coloured volumes are density maps extracted from the simulations, mapping the location of either GND + (blue), the first hydration shell of GND + (red), or the first hydration shell of the carboxylate groups (white). Representative snapshots are shown in Supplementary Fig. 11 . The panel on the right shows the free-energy profile associated with the exchange, as a function of the distances between the GND + ion and S P and S N ( d P and d N ). A two-dimensional free-energy surface is shown in Supplementary Fig. 11 . ( b ) Exchange between the unlocked glutamine side chain in the c 1 subunit (orange sticks) and the glutamate side chain in the adjacent Na + site, counter-clockwise. ( c ) Same as b , clockwise. The c-ring is represented as in Fig. 2 . Hydrogen atoms as well as protein side chains and MPD/water molecules are omitted for clarity. Full size image We next carried out two analogous free-energy simulations in which the GND + ion exchanges between an unlocked glutamate in a c 2/3 subunit and the glutamine in the c 1 subunit, either in the clockwise ( Fig. 8b and Supplementary Fig. 11b ) or counter-clockwise directions ( Fig. 8c and Supplementary Fig. 11c ). Both calculations showed transient binding of GND + to the c 1 glutamine via its carboxamide group. Not surprisingly, the Gln-GND + pair is energetically less favourable than Glu-GND + , but the computed free-energy difference is only ~4 kcal mol −1 (while the barrier between the two states is ~5 kcal mol −1 ). To put this energetic cost in context, note that the necessary release of a bound Na + from the S N site ( Fig. 6 ) entails a free-energy expenditure of ~3 kcal mol −1 (for K d ~0.1 mM and [Na + ] N ~10 mM). Thus, although the formation of the Gln-GND + interaction is likely to slow down the rotary mechanism (see below), this step is not prohibitive from an energetic standpoint. Indeed, a statistical analysis of arginine interactions with ionic and non-ionic side chains in experimental high-resolution protein structures underscores the feasibility of this kind of interaction ( Supplementary Fig. 12 ). Thus, we conclude that the proposed arginine-switch step ( Fig. 6 ) is plausible from an energetic standpoint, both in prototypical F-type rings as well as in A. woodii . Nevertheless, our results indicate that the glutamate-to-glutamine substitution in the V-type c 1 subunit not only precludes Na + binding, but also introduces a non-negligible energetic cost in the dynamic exchange between c-ring/subunit-a interactions. Its impact on the kinetics of c-ring rotation and on the transduction of the sodium-motive force are analysed next. Thermodynamic and kinetic impact of the V-type c-subunit The rotary mechanism of F-, A- and V-type ATPases is a natural consequence of the inherent periodicity of the conformational free-energy landscape of the subunit-a/c-ring complex. Owing to the oligomeric architecture of the c-ring, this landscape consists of a series of resting states, which may interconvert in either direction, stepwise, as ions bind to and become released from the c-ring. The detailed features of this landscape surely vary among different enzymes, but a general implication of the two-channel model described above is that counter-clockwise steps result in ion permeation from the P- to the N-side, and vice versa for clockwise steps. Moreover, when the a/c complex is isolated from the catalytic domain the preferred directionality of these individual steps is determined exclusively by the rates of ion binding from either side of the membrane, that is, by the transmembrane electrochemical gradient. If the c-ring is coupled to F 1 , however, the free energies of ATP synthesis or hydrolysis, which depend on the concentrations of reactants and products (that is, the phosphorylation potential), also contribute to determine the preferred direction of rotation. Excess amounts of ATP will strongly favour hydrolysis and drive the c-ring clockwise, resulting in accumulation of ions on the P-side. By contrast, depletion of ATP, and a sufficient supply of ADP and P i , allows ions to permeate downhill, and the resulting counter-clockwise rotation of the c-ring drives the synthesis and release of ATP. It is in this context that we proceed to analyse the functional implications of the F/V-hybrid ring of the A. woodii ATP synthase, relative to an enzyme with a prototypical c 11 ring. Specifically, we formulated two plausible free-energy landscapes designed to encompass the series of microscopic states and competing processes proposed to underlie the rotary mechanism ( Fig. 9a ); these are largely based on experimental and computational observations, including those reported here. We then used two complementary kinetic-modelling algorithms (Methods) to determine what these energy landscapes imply in regard to the ability of either enzyme to synthesize ATP, driven by an ion gradient, or to create and sustain a gradient, driven by ATP hydrolysis. 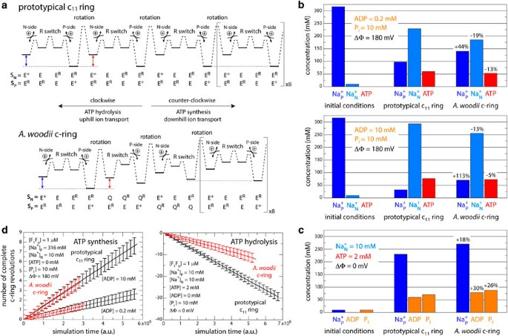Figure 9: Thermodynamic impact of the c1subunit on ATP synthesis and ion transport. (a) Hypothetical free-energy profiles of the c-ring/subunit-a complex, coupled to F1, for a prototypical F-type c11ring with no missing ion-binding sites, and for theA. woodiic-ring. The profiles illustrate the microscopic states, free-energy differences and kinetic barriers employed in the kinetic model of the rotational cycle described in the text. These states are individually identified by the configuration of the SPand SNsites, that is, whether they feature a glutamate (E) or glutamine (Q), whether they are occupied by Na+(E+) or not (E, Q) and whether they are paired with the arginine on subunit-a (ER, QR) (Methods). The profiles shown represent an equilibrium condition in which the sodium-motive force (blue arrow) and the phosphorylation potential (red arrow) are exactly balanced. The simulations are, however, initiated out of equilibrium, that is, the landscapes are heavily tilted in one or other direction, favouring ion-driven ATP synthesis or ATP-driven uphill transport, reaching equilibrium gradually. (b) Production of ATP driven by a variable transmembrane Na+gradient (30-fold initially), under a constant membrane potential of 180 mV, that is, mimicking a voltage-clamp electrophysiological experiment in which the potential is set with K+and valinomycin. The values of [ATP], [Na+]Pand [Na+]Nat equilibrium are compared with those set initially; percentage differences between the values calculated for an ATP synthase with a prototypical c11ring and theA. woodiienzyme are indicated. (c) Generation of a transmembrane Na+gradient, under a constant membrane potential of 0 mV, driven by an excess of ATP over ADP andPi. Equilibrium values for a prototypical c11ring and that inA. woodiiare again compared. (d) Initial rotation rates under the same conditions used inbandc. The data are averages over 100 independent kinetic Monte-Carlo trajectories of 20 million steps each (Supplementary Fig. 13). Figure 9: Thermodynamic impact of the c 1 subunit on ATP synthesis and ion transport. ( a ) Hypothetical free-energy profiles of the c-ring/subunit-a complex, coupled to F 1 , for a prototypical F-type c 11 ring with no missing ion-binding sites, and for the A. woodii c-ring. The profiles illustrate the microscopic states, free-energy differences and kinetic barriers employed in the kinetic model of the rotational cycle described in the text. These states are individually identified by the configuration of the S P and S N sites, that is, whether they feature a glutamate (E) or glutamine (Q), whether they are occupied by Na + (E + ) or not (E, Q) and whether they are paired with the arginine on subunit-a (E R , Q R ) (Methods). The profiles shown represent an equilibrium condition in which the sodium-motive force (blue arrow) and the phosphorylation potential (red arrow) are exactly balanced. The simulations are, however, initiated out of equilibrium, that is, the landscapes are heavily tilted in one or other direction, favouring ion-driven ATP synthesis or ATP-driven uphill transport, reaching equilibrium gradually. ( b ) Production of ATP driven by a variable transmembrane Na + gradient (30-fold initially), under a constant membrane potential of 180 mV, that is, mimicking a voltage-clamp electrophysiological experiment in which the potential is set with K + and valinomycin. The values of [ATP], [Na + ] P and [Na + ] N at equilibrium are compared with those set initially; percentage differences between the values calculated for an ATP synthase with a prototypical c 11 ring and the A. woodii enzyme are indicated. ( c ) Generation of a transmembrane Na + gradient, under a constant membrane potential of 0 mV, driven by an excess of ATP over ADP and P i . Equilibrium values for a prototypical c 11 ring and that in A. woodii are again compared. ( d ) Initial rotation rates under the same conditions used in b and c . The data are averages over 100 independent kinetic Monte-Carlo trajectories of 20 million steps each ( Supplementary Fig. 13 ). Full size image Both these analyses show that ATP synthesis is viable in the A. woodii enzyme, either from a thermodynamic or a kinetic standpoint, in spite of the V-type c-subunit inserted in the c-ring. If, mimicking a voltage-clamp electrophysiological experiment, we initially set a sufficient Na + electrochemical gradient (30-fold) and provide sustained amounts of ADP (2 or 10 mM) and P i (10 mM), the model yields a sizeable ATP output (70 mM) when equilibrium is ultimately reached ( Fig. 9b ). The amount of ATP produced by the A. woodii enzyme, however, is smaller than that synthesized by an equivalent enzyme with a canonical homomeric c 11 ring (5–13% in these conditions), all else being equal ( Fig. 9b ). That is, owing to the missing binding site, the A. woodii enzyme is less able to dissipate the Na + gradient and therefore, from a thermodynamical standpoint, it is a slightly less productive ATP synthase. From a kinetic standpoint, the impact of the V-type c-subunit appears to be small ( Fig. 9d ). As mentioned, the A. woodii model features an additional energetic barrier encountered when the c 1 subunit crosses the a/c interface. However, this barrier is much lower than those limiting the rotation rate when the enzyme functions in synthesis, that is, those associated with the rotational stepping of the c-ring, which are uphill in energy (Methods, equation (10)). Because rotary ATPases are reversible enzymes, these observations raise the question of whether the V-type c-subunit would make the A. woodii enzyme a more capable ion pump than one with a homomeric c 11 ring. The models used above, now examined in conditions that favour ATP hydrolysis, suggest this is indeed the case. If a null electrochemical gradient is initially set, along with sustained ATP and [Na + ] N concentrations (2 and 10 mM, respectively), Na + is progressively accumulated by both enzymes on the P-side of the membrane, as the concentrations of ADP and P i raise ( Fig. 9c ). At equilibrium, however, the Na + gradient built up by the A. woodii ATP synthase (~30 fold) is significantly greater than that produced by the enzyme with a prototypical c 11 ring (18% in these conditions) ( Fig. 9c ). Since the rotational displacements in hydrolysis mode are considerably faster than in synthesis (Methods, equation (11)), the impact of the V-type c-subunit on the overall rotation kinetics is more apparent ( Fig. 9d ), but clearly not critical (~2-fold in our model). In summary, this kinetic-modelling analysis indicates that the impact of the V-type double-hairpin c 1 subunit on the functionality of the A. woodii ATP synthase is not negligible but modest, explaining why this enzyme is the primary source of ATP in this organism. Our analysis also indicates, interestingly, that the V-type c-subunit embedded in the A. woodii c-ring would increase the thermodynamic capacity of the enzyme to generate an ion gradient, if driven by ATP hydrolysis, although this capacity would be maximally realized more slowly than with a prototypical c-ring. Although this observation is not necessarily relevant to the physiology of this acetogenic bacterium, it does have broader implications. By extension, it seems plausible that the evolutionary driving force behind the c-subunit gene duplication and loss of multiple binding sites that is often seen in the rotor rings of eukaryotic V-type ATPases is precisely to maximize the thermodynamic capacity of these enzymes to sustain robust, slowly changing ion gradients, for a limited ATP input, such as those across the membranes of intracellular compartments. The high-resolution crystal structure of the A. woodii c-subunit ring establishes the existence of heteromeric c-rings in the rotary ATPase family and provides unequivocal structural evidence for the Na + dependence of the A. woodii ATP synthase. Moreover, the structure shows that c-subunits with distinct transmembrane topologies and ion-binding site configurations can form functional assemblies. The A. woodii ring consists of nine single-hairpin c-subunits, each harbouring a Na + -binding site, and one double-hairpin c-subunit, with one additional site and one vacancy. Although such heteromeric rotors with missing ion-binding sites are rare in bacteria, they are typical of eukaryotic V-type ATPases, for example, in S. cerevisiae and in humans. To investigate whether such variations might reflect a functional adaptation, we dissected the microscopic rotary mechanism of the A. woodii c-ring via computer simulations and free-energy calculations. The results reveal a mechanism that is largely comparable to that of conventional homomeric c-rings, albeit with slightly altered thermodynamic and kinetic characteristics. In particular, the V-type double-hairpin c-subunit diminishes the extent to which the sodium-motive force may be harnessed for ATP production, but this effect does not appear to be functionally critical. An important related observation of broader implications is that the V-type c-subunit also increases the thermodynamic capacity of the enzyme to create or sustain an electrochemical gradient, relative to an equivalent enzyme with a canonical c-ring of the same size. Such an effect would be amplified if multiple V-type subunits were assembled into the c-ring, as found in vacuolar and plasma-membrane ATPases. Our observations thus suggest that adaptations in the membrane rotor have contributed to the structural–functional evolutionary path from prokaryotic ATP synthases to eukaryotic ATPases. By duplicating the c-subunit genes, the structural stability of the resulting c-rings is actually enhanced, for entropic reasons, thus making the loss of ion-binding sites much more tolerable than for single-hairpin homomeric c-rings. We propose that such adaptations have led to c-ring architectures that are inherently better suited for generation of robust ion gradients than for ATP production. The structure of the A. woodii ring appears to provide a glimpse into this evolutionary path. Cell growth and protein purification A. woodii (DSM 1030) was grown in a 20-l fermenter to an optical density of ~2.5 for ~20 h, as previously described [43] , using 20 mM fructose as carbon source. Washed membrane vesicles [32] were adjusted to a protein concentration of 20 mg ml −1 in buffer A (50 mM Tris/HCl, pH 7.5; 50 mM NaCl; 5 mM MgCl 2 ) and solubilized with 2% (w/v) n -dodecyl-β- D -maltopyranoside for 1 h at 4 °C. The solubilized protein was collected by ultracentrifugation at 350,000 g for 15 min at 4 °C and supplemented with 50 mM MgCl 2 . The ATP synthase was enriched using an ATPase-activity-controlled polyethylene glycol (PEG) precipitation on ice. The 4–10% (w/v) PEG 6000-containing fraction was centrifuged at 8,000 g for 20 min at 4 °C and the ATP synthase-containing pellet was solubilized in buffer B (20 mM Tris/HCl, pH 7.5; 100 mM NaCl; 5 mM EDTA; 0.05% n -dodecyl-β- D -maltopyranoside). For c-ring extraction, the sample was diluted to 5 mg ml −1 , solubilized with 1% (w/v) N -lauroylsarcosine at RT for 1 h, followed by a 10-min incubation at 68 °C. A saturated ammonium sulfate solution (in 50 mM Tris/HCl, pH 8.0) was gradually added to the protein solution up to a 68:32 ratio, respectively, incubated for 20 min at RT and centrifuged at 8,000 g for 20 min. The supernatant was sterile filtered through a 0.2-μm filter (Sarstedt, Nümbrecht, Germany) and dialysed against buffer C (20 mM Tris/HCl, pH 7.5; 50 mM NaCl). The c-ring was further purified using hydroxyapatite (BioGel HT; Bio-Rad, Munich, Germany) and sucrose density gradient centrifugation (5–35% sucrose in 20 mM Tris/HCl, pH 7.5; 50 mM NaCl; 0.1% n -decyl-β- D -maltopyranoside; 220,000 g , 21 h, 10 °C). The sample was dialysed against buffer C for 3 days and concentrated to ~4 mg ml −1 using an Amicon centrifugal filter device with a molecular weight cutoff of 10,000 (Millipore GmbH, Schwalbach, Germany) and stored at 4 °C. 3D crystallization and structure determination Before crystallization, 3% (w/v) n -heptyl-β- D -thioglucopyranoside (Affymetrix GmbH, Munich, Germany) was added to the c-ring sample and incubated overnight at RT, followed by a 10-min incubation at 60 °C and another hour at RT. The protein was mixed in a 1:1 ratio with buffer D (100 mM sodium acetate, pH 4.5; 9% (v/v) PEG 400; 20 mM MnCl 2 ) and crystallization was accomplished using a vapour diffusion hanging drop method in a 24-well plate with 500 μl reservoir (100 mM sodium acetate, pH 4.5; 9% (v/v) PEG 400) at 12 °C in 4 days. After the crystals reached their final size, the PEG 400 concentration was gradually increased from 9 to 40% (v/v) within 48 h and the crystals were flash frozen in liquid nitrogen. Approximately 1,000 crystals were screened at beamlines PX-II X10SA of the Swiss Light Source in Villigen, Switzerland, and ID23.1, ID23.2 and ID29 of the European Synchrotron Radiation Facility in Grenoble, France. The final data set used for this work ( Supplementary Table 1 ) was collected at 100 K at microfocus beamline ID23.2 of the European Synchrotron Radiation Facility. The data were processed using XDS [44] and the structure was determined by molecular replacement with PHASER [45] , using an adapted structure of the c 11 ring from Ilyobacter tartaricus (PDB 1YCE) as a search model. The unit cell, in the P4 3 2 1 2 space group, comprises eight c-rings, with one c-ring as the asymmetric unit ( Supplementary Fig. 4 ). Iterative rounds of model building into the 2 F obs − F calc and F obs − F calc electron-density maps, which were clearly traceable, were carried out with COOT [46] and the resulting model was refined with PHENIX [47] . The final refined structure has no Ramachandran outliers. The final atomic coordinates are deposited in the Protein Data Bank, with accession code 4BEM . AFM and image analysis The unprocessed AFM image used in this study was obtained as described previously [22] and analysed by applying a different classification approach and recent software versions. First, the image was processed using Nanoscope V software (DI–Veeco, Santa Barbara, CA, USA). A gallery of 260 c-rings viewed from the periplasmic side was created in BOXER [48] applying a manual particle-picking procedure and further classification in IMAGIC [49] . Particles were divided into five classes, which are used in the further analysis. 3D representations of the class averages were produced in DINO3D ( http://www.dino3d.org ). Cross-section profiles of the c-ring class averages were created using ImageJ [50] . Other biochemical methods Protein concentrations were determined with the bicinchoninic acid method according to Pierce (Rockford, IL, USA), with BSA as a standard. SDS–PAGE was performed as described previously [51] and all gels were silver stained [52] . ATPase activity was determined by the coupled spectrophotometric assay [53] . Simulation systems and specifications MD simulations were calculated with NAMD 2.7 (ref. 54 ) and the all-atom CHARMM27/CMAP force field [55] , [56] . All simulations were carried out at constant temperature (298 K) and pressure (1 atm) using a Langevin thermostat/barostat, and with periodic boundary conditions. Electrostatic interactions were computed using the particle-mesh Ewald algorithm, with a 12-Å real-space cutoff; van der Waals interactions were truncated also at 12 Å. The c-ring from A. woodii was simulated either in a hydrated 1-palmitoyl-2-oleoyl- sn -glycero-3-phosphocholine (POPC) lipid membrane, or in a solution consisting of MPD and water. The atomic coordinates for the c-ring at the beginning of the simulations were those in the crystal structure at 2.1 Å resolution. The Na + ions and crystallographic water molecules identified in the structure were also included. Both membrane/water and MPD/water systems were prepared as described previously [14] , [57] . The membrane system includes 233 POPC and 18,448 water molecules, in an orthorhombic box 100 × 100 × 95.6 Å. The MPD system includes 750 MPD and 12,363 water molecules, in a cubic box of 86.4 Å, that is, approximately a 30:70 volume ratio. In both systems, nine K + ions were added to neutralize the net charge of the system. After the initial set-up, the protein–lipid and protein–MPD interfaces were equilibrated via simulations of 80 and 200 ns, respectively. During the equilibrations, the dynamics of the c-ring was restricted using a combination of position, distance and conformational restraints, which were gradually released. Simulations of spontaneous Na + unbinding and rebinding To characterize the dynamics of the c-ring and study the mechanism of Na + unbinding, two unrestrained simulations of 350 ns each were calculated for the MPD system and one simulation of 260 ns was calculated for the POPC system. Both MPD simulations revealed Na + dissociation events. A third simulation of 200 ns was also calculated to study the mechanism of Na + rebinding. This last simulation was initiated 45 ns after one of the Na + dissociation events, when the unbound Na + approached the c-ring binding site (within 25 Å) from which it originated, after diffusing across the simulation box. To preclude the ion from diffusing away from the c-ring, a harmonic soft-wall ( k =15 kcal mol −1 Å −2 ) was introduced, at a distance of 20 Å from the carboxylic group (Glu62) that coordinates the ion in the binding site. This confinement effect is equivalent to that of a ~100 mM NaCl concentration and does not interfere with the ion–protein interaction. Additional simulations of the c-ring in MPD/water were prepared to assess whether the c 1 subunit may bind Na + in a hydrophilic environment. Na + was modelled into this site in a hypothetical coordination network optimized through a 5-ns simulation with ion–protein distance restraints, namely to Gln129(Oε1), T80(Oγ) and V77(O) (each restraint consisted of a harmonic potential flat-bottomed up to 3 Å and with k =15 kcal mol −1 Å −2 ). Five independent simulations were then carried out without restraints. Free-energy calculations A series of enhanced-sampling MD simulations of the c-ring in MPD/water were designed to gain insights into the energetics of two key elements in the proposed rotary mechanism. First, to assess the putative role of a conserved arginine in TM4 of subunit-a in precluding direct ion hopping between the two binding sites at the a/c interface, we extracted a snapshot from one of the unbiased simulations of the c-ring in MPD/water after a spontaneous Na + unbinding event, and the exposed Glu62 side chain in the empty site was allowed to form an ion pair with a guanidinium cation (GND + ) added to the buffer. The free-energy cost of transferring a Na + ion to this unlocked, GND + -paired site from an adjacent locked binding site was then computed using the Free-Energy Perturbation method [54] . To model the configuration of the unlocked, GND + -paired site bound to Na + , we used the same procedure described above for the c 1 subunit. The transfer free energy was evaluated in both directions, using a decoupling/re-coupling scheme comprising 40 intermediates. Each intermediate simulation consisted of a 100-ps equilibration followed by 1 ns of averaging time. The GND + -carboxyl ion pair was maintained using a distance restraint (a harmonic potential flat-bottomed up to 3.8 Å and with k =15 kcal mol −1 Å −2 ); the effect of this restraint on the transfer free energy value is<0.1 kcal mol −1 . Free-energy calculations were also used to evaluate the plausibility of the proposed switch of interactions between the subunit-a arginine and either of the two c-ring binding sites exposed to the a/c interface (when both are concurrently ion free). The c-ring was prepared in three configurations, namely (a) with two adjacent binding sites in c 2/3 /c 2/3 interfaces in the ion-free state, (b) with the binding site in the c 1 /c 2/3 interface in the ion-free state and (c) with the binding site in the c 2/3 /c 1 interface in the ion-free state. A GND + cation was again added to the MPD/water buffer in all systems and allowed to form an ion pair with one of the exposed Glu62 side chains. The Adaptive Biasing Force method [58] was then used to simulate the reversible exchange of GND + interactions with (a) either of the two ion-free c 2/3 /c 2/3 binding sites, (b) the ion-free c 2/3 /c 1 site and the c 1 site, and (c) the c 1 site and the ion-free c 2/3 /c 1 site. Two reaction coordinates were employed to bias the sampling in these simulations, namely the distances between the centres-of-mass of GND + and the carboxylate/carboxamide groups of the glutamate/glutamine side chains in the c-subunits involved. The range of distances explored was 3–18 Å. The diffusion of the GND + ion in the direction perpendicular to the membrane plane was confined to a region 10 Å in width, centred at the binding sites. Two-dimensional and one-dimensional free-energy landscapes were obtained from each of these simulations, which lasted (a) 150 ns, (b) 280 ns and (c) 280 ns, respectively. The sampling of the landscape was carried in bins of 0.25 Å for each reaction coordinate; at each bin, 1,000 samples were collected before applying the biasing force. Kinetic model of the coupled F 1 F o enzyme A kinetic model was designed to evaluate the influence of the c 1 subunit on the thermodynamic capacity and rotation rate of the A. woodii ATP synthase under conditions that favour either ATP synthesis, driven by downhill ion permeation, or ATP hydrolysis, resulting in the generation of an ion gradient. The results were compared with an analogous model for a canonical F-type homomeric c-ring with 11 subunits and no missing binding sites. Both kinetic models are based on the premise that the rotation of the c-ring can be described by a series of discrete rotational states Ω i , each of which is uniquely defined by the two specific c-subunits that are concurrently exposed to subunit-a, denoted by S P , S N ; all other sites, denoted by S M , face the lipid membrane. Therefore, the 11 rotational states of the a/c complex would be: Note that this specific numbering reflects counter-clockwise rotations. Also note that the model allows transitions between adjacent rotational states only, and thus state Ω 11 is followed/preceded by Ω 1 . In addition, we postulate that each of these rotational states comprises the series of sub-states depicted in Fig. 6 . Specifically, ion-binding sites (that is, those featuring a glutamate residue) exposed to the membrane (S M ) are assumed to be locked in the Na + -bound state (E + ), while those exposed to subunit-a (S P , S N ) are either Na + -bound (E + ), Na + -free (E) or engaged to the key arginine side chain in subunit-a (E R ). In the A. woodii model, the site within the c 1 subunit is always Na + -free (Q), but it can also engage the arginine in subunit-a (Q R ). The connectivity between these sub-states is pre-defined (according to Fig. 6 ), but all transitions are reversible. A partial sequence of sub-states for the A. woodii model is, for example (the two c-subunits at S P and S N are again indicated in bold): The profiles shown in Fig. 9a represent graphically the relative free-energy values and kinetic barriers between these rotational states and sub-states; these reflect available experimental measurements and MD simulation data, and also account for the effect of the sodium-motive force and the phosphorylation potential. Specifically, the energy cost of Na + unbinding from the S N site is: where Δ G b ~ −5.5 kcal mol −1 is the standard Na + binding affinity at pH 7 (unpublished experimental results) and [Na + ] N is the Na + concentration on the N-side of the membrane. ΔΨ is the electrostatic potential applied across the membrane (as in a voltage-clamp experiment), F and k B are the Faraday and Boltzmann constants and T the temperature (300 K). Similarly, the free-energy gain associated with Na + binding to the S P site is: Based on the free-energy simulations summarized in Fig. 8 , for the arginine-switch step: Lastly, each rotational step entails a free-energy cost in the counter-clockwise direction (or gain, if clockwise), due to the mechanical coupling between the c-ring and the catalytic domain: where Δ G 0 ~ −7.3 kcal mol −1 is the standard free energy of ATP hydrolysis at pH 7 (ref. 59 ). Note that the assumption implicit in equation (5) is that the cost or gain associated with ATP synthesis or hydrolysis is uniformly distributed over all rotational steps; this is consistent with the notion of an elastic transmission between the F 1 and F o domains [60] . The relative free-energy values defined in equations (1, 2, 3, 4, 5) determine the transition rates between adjacent sub-states in the rotational cycle [61] . For example, for Na + unbinding from and rebinding to the S N site, these rates are, respectively: Note only the latter is dependent on [Na + ] N . Likewise, for the S P site: And for the transition between rotational steps: Note that the rate of counter-clockwise rotations (equation (10)) is accelerated by [ADP] and [P i ], while that of clockwise rotations (equation (11)) is enhanced by [ATP]. The exponential pre-factors κ and κ ’ in equations (6, 7, 8, 9, 10, 11) can be thought as the intrinsic transition rates in the absence of a driving force. For simplicity, we used κ =1, and κ ′=10 −6 , that is, the assumed kinetic barrier between rotational states is effectively ~8 kcal mol −1 greater than for between sub-states. We believe this assumption is justified given that rotational transitions involve a large-scale reconfiguration of the c-ring interface with both subunit-a and the lipid membrane, and possibly a conformational change within subunit-a as well. By contrast, transitions between sub-states entail only structurally localized changes, coupled to the exchange of Na + with the bulk solution, which are likely to be kinetically faster under physiological conditions. Two complementary algorithms were used to characterize the multi-state kinetic model just described. In the first algorithm, initial concentration conditions are set for Na + , on either side of the membrane, and for ATP, ADP and P i , and system of interdependent differential equations describing the time evolution of all species in the model is resolved so as to determine the concentrations of at equilibrium [62] . That is, the model predicts how the thermodynamic driving forces associated with an initial chemical imbalance are transduced to yield one or other output, leaving aside kinetic effects. In the second approach, the time evolution of the rotary mechanism is explicitly analysed, for the same out-of-equilibrium initial conditions, using a kinetic Monte-Carlo algorithm [63] . To do so, the cycle is initiated in a sub-state chosen at random, and evolved through a stochastic, iterative procedure, according to the instantaneous probability a forward or a backward transition, P + or P − . These probabilities are derived from the set of rates defined in, for example, equations (6, 7, 8, 9, 10, 11), that is,: To determine whether the cycle proceeds forward or backward at a given time, a random number R uniformly distributed between 0 and 1 is generated at each iteration; if R < P + , the cycle evolves forward and otherwise backward. Either way, the simulated time increases by: where r is also a random number uniformly distributed between 0 and 1 generated at each iteration. The outcome of this iterative procedure is a rotational stochastic trajectory. Initially, these trajectories reflect a preferential directionality, but at equilibrium clockwise and counter-clockwise rotations balance each other. How to cite this article : Matthies, D. et al . High-resolution structure and mechanism of an F/V-hybrid rotor ring in a Na + -coupled ATP synthase. Nat. Commun. 5:5286 doi: 10.1038/ncomms6286 (2014). Accession codes: Coordinates and structure factors have been deposited at the Protein Data Bank with the accession code 4BEM .